TRPV channel-mediated calcium transients in nociceptor neurons are dispensable for avoidance behaviour Animals need to sense and react to potentially dangerous environments. TRP ion channels participate in nociception, presumably via Ca 2+ influx, in most animal species. However, the relationship between ion permeation and animals’ nocifensive behaviour is unknown. Here we use an invertebrate animal model with relevance for mammalian pain. We analyse the putative selectivity filter of OSM-9, a TRPV channel, in osmotic avoidance behaviour of Caenorhabditis elegans . Using mutagenized OSM-9 expressed in the head nociceptor neuron, ASH, we study nocifensive behaviour and Ca 2+ influx. Within the selectivity filter, M 601 -F 609 , Y604G strongly reduces avoidance behaviour and eliminates Ca 2+ transients. Y604F also abolishes Ca 2+ transients in ASH, while sustaining avoidance behaviour, yet it disrupts behavioral plasticity. Homology modelling of the OSM-9 pore suggests that Y 604 may assume a scaffolding role. Thus, aromatic residues in the OSM-9 selectivity filter are critical for pain behaviour and ion permeation. These findings have relevance for understanding evolutionary roots of mammalian nociception. Since their discovery in fly phototransduction, transient receptor potential (TRP) ion channels have been found to critically function in neurosensory transduction across phyla except in plants and bacteria [1] , [2] . They have a role in several sensory submodalities, including osmotic, thermal, mechanical, photo (including ultraviolet radiation) and acid sensing [3] , [4] , [5] , [6] , [7] , [8] , [9] , [10] , [11] , [12] . Of particular medical importance, they have a role in pain transduction [7] , [13] , [14] , [15] . The TRP superfamily of ion channels comprises the TRPC, TRPN, TRPY, TRPV, TRPM, TRPP, TRPML and TRPA subfamilies, all of which are characterized by intracellular N and C termini, six transmembrane segments (TM1–TM6), and a pore loop connecting TM5 and TM6 (ref. 16 ). TRP channels (TRPCs) are arranged in a homo- or hetero-tetrameric manner, around an ion-conducting pore, analogous to that of voltage-gated potassium (Kv) channels [17] . Similar to Kv channels, TRPCs are postulated to possess an ion selectivity filter. For all Kv channels, permeation is controlled by a series of amino acids C-terminal to the pore helix before the final TM domain [18] , [19] . Mutational, biophysical and computational analysis revealed that the critical region for ion selectivity is a conserved series of residues with the following properties: TXXTXGYG [20] . With the landmark determination of the KcsA crystal structure, the importance of the selectivity filter and the properties of the signature residues were confirmed and expanded to new levels [21] . The process of permeation and ion selectivity has been investigated in TRPCs using heterologous cellular expression systems, with the most well-investigated subfamilies being TRPV and TRPM [17] , [22] , [23] . Of note, both subfamilies have been linked to pain signalling and are known to conduct Ca 2+ (refs 5 , 15 , 24 , 25 ). Most of these channels show an increased selectivity for Ca 2+ over Na + (refs 1 , 16 , 26 , 27 , 28 ), presumably as a function of the selectivity filter. In sharp contrast to the pivotal relevance of the selectivity filter for the biophysical function of the channel, as established by cellular studies, investigations of the presumed selectivity filter region in live animals are largely missing. Of particular note is the lack of research into the effect of TRPC-mediated Ca 2+ influx on animal behaviour. Studies that focus on the function of the TRPC selectivity filter would help us to better understand which residues are critical for ion permeation and selectivity in live animals as they respond to (noxious) external cues. The C. elegans TRPV ion channel, OSM-9, is the functional homologue of mammalian TRPV4 and functions in signal transduction in response to noxious osmotic, volatile chemical and mechanical cues [29] , [30] . The role of TRPV4 in pain signalling has become increasingly clear by accumulating experimental evidence for over a decade [5] , [7] , [11] , [13] , [15] , [29] , [31] , [32] , [33] . In worms, both OSM-9 and its partner TRPV channel, OCR-2, are expressed throughout the soma, dendrite and sensory cilia of the ASH head nociceptor neuron. The sensory cilium of this neuron directly interfaces with the external environment. Both OSM-9 and OCR-2 are required for ASH-mediated avoidance behaviour [34] , [35] . Systematic study of avoidance behaviour in invertebrates can be used for elucidating nocifensive signalling and neural circuitry. Thus, studies of invertebrate nocifensive behaviour can provide useful guidance to study pain mechanisms in ‘higher’ animals with the distinct advantage of facilitated discovery of inherent genetic mechanisms [30] , [36] . Mechanisms of ASH activation are not completely understood, although Ca 2+ influx is postulated to have a major role. It is known that the genes osm-9 , ocr-2 and egl-19 (the only C. elegans L-type voltage-gated calcium channel) are required for Ca 2+ influx into ASH [37] . It has been implied that OSM-9 is conducting Ca 2+ when worms encounter noxious stimuli, but this has not been addressed experimentally. As mentioned above, while TRP(V) channels have been studied to elucidate ionic permeation and selectivity by relying on heterologous cellular systems, very few channels have been examined using in vivo techniques. Only two such studies investigated TRP selectivity filters in vivo . Liu et al. [38] demonstrated that the Drosophila TRP channel (dTRP; TRPC) is a pore forming channel subunit, that residue D 621 within the selectivity filter of dTRP is responsible for Ca 2+ permeation into fly photoreceptors, and that Ca 2+ is essential for phototransduction in photoreceptor cells and their survival. In a landmark paper, Kang et al. [39] showed that C. elegans TRP-4, a TRPN subfamily member, is a mechanotransduction channel, functional in sensing of external viscosity, and that mutations in the predicted selectivity filter region are critical for channel functioning. In the present study, we set out to examine the structure–function relationship of OSM-9, using the well-characterized osmotic avoidance behaviour as a readout of nocifensive behaviour [40] , [41] . Specifically, we wanted to determine whether OSM-9 is a pore-forming subunit of an ion channel that conducts Ca 2+ , and investigate which amino acids C-terminal to the pore helix might contribute to its Ca 2+ selectivity properties. Our systematic approach analyses nocifensive behaviour for multiple noxious stimuli (osmolarity, volatile chemicals and mechanical), Ca 2+ influx into ASH in live worms and high-powered microscopy to verify expression of the transgenes in the sensory cilia of the ASH head nociceptor neuron and proper interaction of the OSM-9 channel isoforms with their partner TRPV channel, OCR-2. In addition, our approach is complemented by computational modelling and molecular dynamic refinement of the OSM-9 channel structure. Taken together, our results suggest that OSM-9 functions as an ion channel in vivo , and that negative and aromatic residues within the selectivity filter are critical for worm nocifensive behaviour and Ca 2+ influx into the ASH head nociceptor neuron. Most novel to us were the findings that avoidance behaviour can be sustained in the absence of measurable Ca 2+ transients in the nociceptor neuron, yet we also noticed that behavioral plasticity was attenuated in this case. OSM-9 residues that are critical for osmotic avoidance behaviour Sequence alignments of mammalian TRPV channels with the bacterial Kv channel, KcsA, show that these channels share sequence similarity within the region of the selectivity filter (selectivity filter: percentage identity, 42.9% (seven residues), Supplementary Fig. 1 ) [16] . In heterologous cellular expression systems, mutation of negatively charged residues in the respective region of TRPV1 and TRPV4 have resulted in altered selectivity and reduced permeation of divalent cations, specifically Ca 2+ and Mg 2+ (refs 26 , 28 ). Against this background, we investigated the residues C-terminal to the pore helix of OSM-9. We interrogated their role in activation of, and Ca 2+ influx into, ASH and their impact on nocifensive behaviour ( Supplementary Note 1 ). We focused on those residues that followed the presumed pore helix of OSM-9 (ref. 42 ). OSM-9 protein domains were confirmed by redundant computational analyses ( Supplementary Fig. 2 ). We first deleted groups of six residues across the entire loop 6 region ( Fig. 1a ). We found that the first and second deletions had the strongest effects on osmotic avoidance behaviour ( Supplementary Note 1 ), so we focused our studies on this subdomain ( Fig. 1b ). We next deleted groups of three amino acids ( Fig. 1c ) and exchanged the first nine individual amino acids with alternate residues ( Fig. 1d ). Behavioral analysis of these mutants showed that residues 601 MGG 603 and 604 YDY 606 have the most significant impact on osmotic avoidance. The observed responses varied from nearly wild type (WT) to almost completely defective for the individual exchanges. We divided our scoring into categories of behaviour based on the average avoidance index obtained for each strain (see Methods section). Those that fell between 0.0 and −0.25 were termed WT responders, −0.26 to −0.74 were termed partially defective and −0.75 to −1.0 were termed defective. 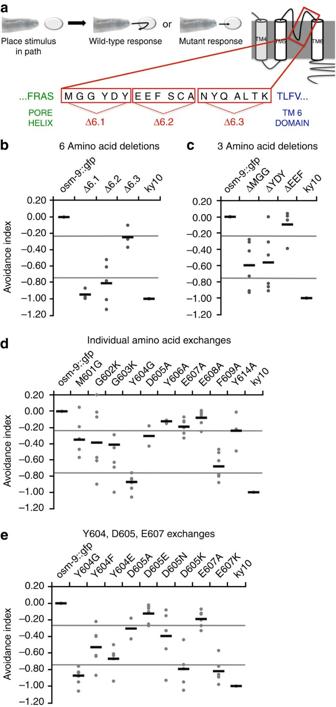Figure 1: OSM-9 mutations result in avoidance defects mediated by ASH (a) Schematic of worm avoidance behaviour and loop 6 sequence of OSM-9. A quantity of 1 M fructose is dropped in the pathway of a forward-moving worm. WT worms swiftly reverse the direction after touching the aversive liquid, whereas mutant worms continue moving forward through the drop after contact. Schematic of OSM-9 protein structures and sequence C-terminal to the pore helix, before TM6, depicting orientation of 6 and 3 amino acid deletions. (b–e) Behavioral avoidance metrics for amino acid deletions and exchanges in OSM-9. Percent avoidance is acquired by averaging number of responders divided by number of animals tested from 5 to 6 worms per transgenic line, from each of three lines to give a total of 15–18 worms tested. Percent avoidance for each strain is normalized toosm-9::gfpWT rescue andosm-9 (ky10)strain values for the time point it was collected. This process is completed twice and values are averaged to produce the avoidance index. Strains with an avoidance index ≥−0.25 are considered WT, between −0.26 and −0.74 are considered partially defective, and ≤−0.75 are considered defective. Black lines represent mean of the grey dots, each grey dot represent results from 10 individual animals on a given day of testing. Each strain had three independent lines that were tested on 2 separate days. Figure 1: OSM-9 mutations result in avoidance defects mediated by ASH ( a ) Schematic of worm avoidance behaviour and loop 6 sequence of OSM-9. A quantity of 1 M fructose is dropped in the pathway of a forward-moving worm. WT worms swiftly reverse the direction after touching the aversive liquid, whereas mutant worms continue moving forward through the drop after contact. Schematic of OSM-9 protein structures and sequence C-terminal to the pore helix, before TM6, depicting orientation of 6 and 3 amino acid deletions. ( b – e ) Behavioral avoidance metrics for amino acid deletions and exchanges in OSM-9. Percent avoidance is acquired by averaging number of responders divided by number of animals tested from 5 to 6 worms per transgenic line, from each of three lines to give a total of 15–18 worms tested. Percent avoidance for each strain is normalized to osm-9::gfp WT rescue and osm-9 (ky10) strain values for the time point it was collected. This process is completed twice and values are averaged to produce the avoidance index. Strains with an avoidance index ≥−0.25 are considered WT, between −0.26 and −0.74 are considered partially defective, and ≤−0.75 are considered defective. Black lines represent mean of the grey dots, each grey dot represent results from 10 individual animals on a given day of testing. Each strain had three independent lines that were tested on 2 separate days. Full size image We found that Y604G mutants were completely defective, and M601G, G602K, G603K and D605A were partially defective ( Fig. 1d ). Y606A, E607A and E608A mutants were WT responders ( Fig. 1d ), and F609A mutants were partially defective, bordering on defective. We also assessed whether the most severe of these mutations, Y604G, affected additional sensory submodalities of OSM-9 by testing for volatile chemical and mechanical avoidance. We found greatly reduced function for all submodalities ( Supplementary Fig. 3 ). Using avoidance behaviour as a readout for ASH activation and OSM-9 channel function, we conclude that the OSM-9 selectivity filter covers amino acids 601–609, with critical contribution of the first five residues, M 601 -D 605 plus F 609 . Following these studies, we performed a more in-depth analysis of the function of residue Y 604 . To determine which properties of Y 604 were most critical for in vivo channel function, we exchanged it with residues that have similar properties, phenylalanine (F) and glutamic acid (E). Tyrosine is a large residue that can contribute to hydrogen bonding and act in scaffolding of proteins. By comparison, phenylalanine also has aromatic properties, but is non-polar and cannot offer an –OH group to a hydrogen bond. Glutamic acid is a negatively charged amino with a relatively large side chain. Interestingly, we found that Y604F partially rescued the defects observed in Y604G, but it did not rescue the defect to WT levels. Y604E did not significantly rescue the defects, indicating that replacement with a large side-chain amino acid that can possibly provide a favourable charge landscape of the selectivity filter for permeation of cations does not suffice. Taken together, these findings indicate that aromaticity is critical at position Y 604 for the proper function of the selectivity filter in OSM-9. Interested in a possible trend, we evaluated residue Y 606 in a similar manner, leading us to conclude that aromaticity is not critical at this position, as illustrated by WT avoidance behaviour of the Y606A mutation ( Fig. 1d ). For Y604F worms, we also characterized their volatile chemical avoidance and detected a partial rescue, in keeping with osmotic avoidance ( Supplementary Fig. 2 ). To complement the in-depth studies of residue Y 604 , we carried out a similar approach with negatively charged amino acids, D 605 and E 607 . We exchanged D 605 with glutamic acid (E), asparagine (N) and lysine (K). Aspartic acid is a negatively charged, hydrophilic residue. Glutamic acid is also a negatively charged residue that can replace aspartic acid, whereas asparagine is also a hydrophilic residue, but neutral in charge. Lysine is positively charged and hydrophilic. We found that D605K was highly defective, D605E was WT and D605N was only partially defective ( Fig. 1e ). These results led us to conclude that negative charge at position 605 is critical to osmotic avoidance behaviour. In extension, charge reversal via E607K also resulted in highly defective avoidance behaviour ( Fig. 1e ). D605K was also highly defective for the mechanical and chemical submodalities for eliciting avoidance behaviour ( Supplementary Fig. 3 ). Taken together, these findings define the critical region of the selectivity filter to be residues M 601 -D 605 , plus E 607 and F 609 . Loop 6 mutations do not result in altered OSM-9 expression High-powered confocal imaging revealed that OSM-9::GFP is localized to the cilium of the ASH neuron, and can be seen in the soma and occasionally in the dendrite ( Fig. 2a–l ). Analysis of individual amino acid exchanges showed that all mutant proteins are expressed properly in the ASH soma in 85–100% of observed animals and localized to the cilia in 60–95% of animals. The data for each strain tested are summarized in Table 1 . 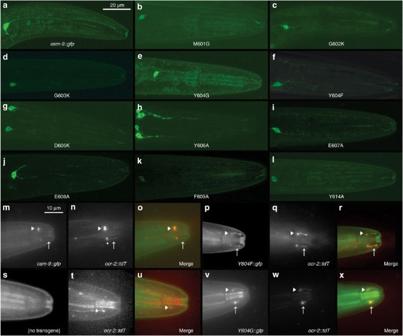Figure 2: Expression analysis of WT, mutant OSM-9::GFP and OCR-2::tdT (a–l) Representative confocal images of transiently expressed WT and mutant OSM-9::GFP protein in the cilium and soma of ASH. All transgenes were expressed inosm-9(ky10)mutant background. (m–x) Representative Delta Vision images of OCR-2::tdT and OSM-9::GFP co-localization in ASH neurons ofosm-9(ky10)worms. Tomato (tdT) fluorescence is significantly stronger than standard GFP and has been reduced in many images. Red and green channels are displayed separately in grey scale to overcome background autofluorescence and better visualize cilia. White arrows mark ciliary expression and arrow heads mark expression in the ciliary transition zone between dendrite and cilium. (S-U)OCR-2::tdTexpression inosm-9(ky10)background. No ciliary expression is apparent in the green or red channel, butOCR-2::tdTappears localized to the ASH dendrite and ciliary transition zone. To compensate for reducedOCR-2::tdTexpression in theosm-9(ky10)background, brightness in the red channel has been increased to visualize the dendrite–ciliary transition zone. More than six experimental repetitions per strain were conducted for each microscopy method, confocal and Delta Vision. Figure 2: Expression analysis of WT, mutant OSM-9::GFP and OCR-2::tdT ( a – l ) Representative confocal images of transiently expressed WT and mutant OSM-9::GFP protein in the cilium and soma of ASH. All transgenes were expressed in osm-9(ky10) mutant background. ( m – x ) Representative Delta Vision images of OCR-2::tdT and OSM-9::GFP co-localization in ASH neurons of osm-9(ky10) worms. Tomato ( tdT ) fluorescence is significantly stronger than standard GFP and has been reduced in many images. Red and green channels are displayed separately in grey scale to overcome background autofluorescence and better visualize cilia. White arrows mark ciliary expression and arrow heads mark expression in the ciliary transition zone between dendrite and cilium. (S-U) OCR-2::tdT expression in osm-9(ky10) background. No ciliary expression is apparent in the green or red channel, but OCR-2::tdT appears localized to the ASH dendrite and ciliary transition zone. To compensate for reduced OCR-2::tdT expression in the osm-9(ky10) background, brightness in the red channel has been increased to visualize the dendrite–ciliary transition zone. More than six experimental repetitions per strain were conducted for each microscopy method, confocal and Delta Vision. Full size image Table 1 OSM-9 expression in ASH head nociceptor neurons. Full size table Given the importance of documenting that mutant OSM-9 channel proteins are properly targeted to the ASH cilia, we also designed a complementary functional assay to assess ciliary trafficking. For this assay, we took advantage of the established mechanism that OSM-9 requires its partner TRPV channel OCR-2 for proper ciliary localization [36] . Using the construct sra-6 p:: ocr-2::tdT (tomato), we tested whether mutant OSM-9::GFP was capable of localizing OCR-2::tdT to the cilia. This was accomplished by observing the expression and co-localization of red tomato- and green GFP fluorescence, taking advantage of high-powered deconvolution microscopy. We recapitulated functionality of this assay because GFP and tomato co-localization was observed in 100% in the cell body of ASH and 92% in the cilia for the osm-9::gfp WT rescue strain. Furthermore, tomato fluorescence was observed 100% in the cell body of ASH and 0% in the cilia of the osm-9(ky10) mutant ( Fig. 2m–x ). Co-expression of OCR-2::tdT and OSM-9 mut ::GFP was observed in the cilia of animals expressing OSM-9 mutations in 52–98%, corroborating the confocal data. Details for all mutant strains analysed are summarized in Fig. 2m–x and Table 2 . Table 2 OCR-2 and OSM-9 co-expression in ASH head nociceptor neurons. Full size table For both imaging methods used, visible protein expression was weak for certain strains, specifically for strains that exhibited WT levels of osmotic avoidance. Expression of OSM-9 and OCR-2 protein is known to be in low abundance [36] , so that low-level expression is difficult to visualize over background autofluorescence in the cilia. Protein expression levels may explain why visualized fluorescence did not amount to >90% for each strain tested. This is exemplified by Y606A mutants that exhibited properly localized protein in only 59% of cilia, but showed WT levels of behavioral avoidance. Conversely, D605K mutants exhibited properly localized protein in 95%, but were completely defective in osmotic avoidance. Importantly, when viewing both imaging methods and behaviour together, their combined results suggest strongly that the behavioral defects observed in transgenic strains with mutated OSM-9 channels are not due to defects in localization, but rather due to non-functional channels expressed in the cilia. Residues necessary for proper Ca 2+ entry into ASH via OSM-9 To determine whether the selectivity filter residues 601–609 contributed to Ca 2+ entry into ASH, we conducted in vivo Ca 2+ imaging with worms transgenically co-expressing the Ca 2+ indicator protein, G-CaMP3 and mutated OSM-9 channel proteins, both directed to the ASH nociceptor neuron by use of the sra-6 promoter. These transgenic worms were subjected to noxious osmotic cues in the ‘olfactory chip’, a microfluidics device that allows for controlled exposures of confined, live worms. Animals were stimulated with 1 M fructose [43] . All mutant strains were assessed for their ASH Ca 2+ transients. Hallmarks of a WT response include the ON response (a Ca 2+ spike shortly after stimulus addition), plateau of the Ca 2+ signal and the OFF response (a second Ca 2+ peak after stimulus removal). A WT Ca 2+ transient for the osm-9::gfp WT rescue strain, averaged from 14 responses, is shown in Figs 3 and 4a and Supplementary Figs 4–7 . As a negative control, osm-9(ky10) null animals were imaged in the same manner resulting in a complete lack of change of the Ca 2+ trace ( Figs 3 and 4 ). These experiments were also carried out with glycerol as an osmotic stimulus, leading to similar results for the controls as were recorded with fructose (results not shown). 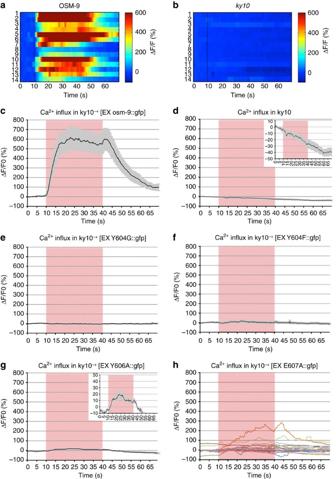Figure 3: Point mutations in OSM-9 alter Ca2+transients in ASH (a,b) Heat maps forosm-9::gfpWT rescue andosm-9 (ky10)worms, depicting all worms tested for each genotype. Trial number is on the left axis and pseudo colour index is shown on the right axis. (c–f) Average Ca2+transients in ASH neurons ofosm-9(ky10)worms transiently expressing WT and mutant OSM-9::GFP. Averages are generated from 12 to 16 animals for each strain, where each animal is stimulated and analysed once. All transients are displayed as ΔF/F of G-CaMP (see Methods section). (a)osm-9::gfpWT rescue strain displays a WT Ca2+transient. (c,d) Y604G and Y604F Ca2+transients are flat and resemble that ofosm-9(ky10)animals. (e) Y606A mutants display reduced Ca2+transients in those animals that respond to stimuli, inset displays 10-fold reduced scale and resulting Ca2+transient. (f) E607A mutant animals display altered Ca2+dynamics. Raw data are displayed, so as not to lose inconsistencies in the individual trials. Figure 3: Point mutations in OSM-9 alter Ca 2+ transients in ASH ( a , b ) Heat maps for osm-9::gfp WT rescue and osm-9 (ky10) worms, depicting all worms tested for each genotype. Trial number is on the left axis and pseudo colour index is shown on the right axis. ( c – f ) Average Ca 2+ transients in ASH neurons of osm-9(ky10) worms transiently expressing WT and mutant OSM-9::GFP. Averages are generated from 12 to 16 animals for each strain, where each animal is stimulated and analysed once. All transients are displayed as ΔF/F of G-CaMP (see Methods section). ( a ) osm-9::gfp WT rescue strain displays a WT Ca 2+ transient. ( c , d ) Y604G and Y604F Ca 2+ transients are flat and resemble that of osm-9(ky10) animals. ( e ) Y606A mutants display reduced Ca 2+ transients in those animals that respond to stimuli, inset displays 10-fold reduced scale and resulting Ca 2+ transient. ( f ) E607A mutant animals display altered Ca 2+ dynamics. Raw data are displayed, so as not to lose inconsistencies in the individual trials. 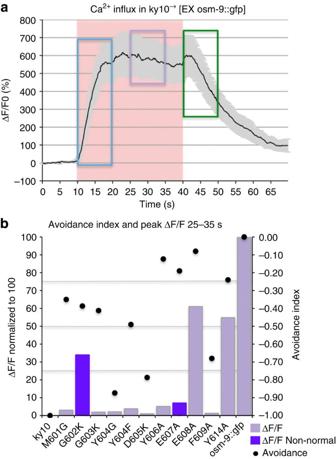Figure 4: Summary of Ca2+imaging and avoidance behaviour (a) WT Ca2+transient obtained from OSM-9::GFP. The distinct phases of the Ca2+transient are noted on the transient. The ON response peak is highlighted in blue, the plateau is highlighted in purple and the OFF response is highlighted in green. (b) The average peak value from the plateau period is shown, after normalization to OSM-9::GFP. Avoidance index (dots) is plotted together with average peak height of the Ca2+transient from the plateau phase for each OSM-9 mutant. Bars in purple refer to values that were derived from averaging of non-normal data sets. Avoidance index is displayed on the right and average peak height of the Ca2+transient is displayed on the left. Note that only two mutants, Y604G and D605K display both, defective osmotic avoidance behaviour and absence of an appreciable Ca2+transient, thus both representing ‘dead channels’. Full size image Figure 4: Summary of Ca 2+ imaging and avoidance behaviour ( a ) WT Ca 2+ transient obtained from OSM-9::GFP. The distinct phases of the Ca 2+ transient are noted on the transient. The ON response peak is highlighted in blue, the plateau is highlighted in purple and the OFF response is highlighted in green. ( b ) The average peak value from the plateau period is shown, after normalization to OSM-9::GFP. Avoidance index (dots) is plotted together with average peak height of the Ca 2+ transient from the plateau phase for each OSM-9 mutant. Bars in purple refer to values that were derived from averaging of non-normal data sets. Avoidance index is displayed on the right and average peak height of the Ca 2+ transient is displayed on the left. Note that only two mutants, Y604G and D605K display both, defective osmotic avoidance behaviour and absence of an appreciable Ca 2+ transient, thus both representing ‘dead channels’. Full size image Of the mutants that exhibited defective osmotic avoidance behaviour, we found that Y604G and D605K displayed flat Ca 2+ transients, suggesting the elimination of channel function, in accordance with their lack of avoidance behaviour for all submodalities ( Figs 3e,f and 4b and Supplementary Fig. 3 ). We were not surprised by the results of the D 605 charge reversal [38] . The lack of Ca 2+ influx in these mutants is in keeping with their impact on nocifensive behaviour, confirming and extending their critical relevance for OSM-9 selectivity filter function in vivo . We remain aware of the limitation of our Ca 2+ imaging method to demonstrate and resolve local Ca 2+ dynamics where ASH connects with the next neuron in the circuit directing avoidance behaviour. One view is that synaptic vesicle released here depends on Ca 2+ influx via voltage-gated channel UNC-2 (ref. 44 ), an alternate view is centred around gap junction-mediated coupling from ASH to the next neuron [45] , [46] . However, these exciting alternate mechanisms for circuit activation will be suitable subjects for future studies and do not subtract from the value of our transduction-focused study presented here. ASH Ca 2+ transients are dispensable for nocifensive behaviour Not expected, against a background of previous evidence and conceptual reasoning of TRP ion channel function in pain signalling/nociception [17] , [47] , [48] , [49] , [50] , [51] , [52] , we found that when compared with the osm-9::gfp WT rescue strain, all mutants exhibited significantly altered Ca 2+ dynamics, except for E608A and Y614A, the latter an aromatic mutation likely outside the selectivity filter ( Supplementary Fig. 5F ). Also, presence of intact Ca 2+ transients in E608A and Y614A mutations lends additional credence to the findings of altered Ca 2+ dynamics in all other selectivity filter mutations. These provocative results suggest strongly that nocifensive behaviour in response to osmotic cues does not fully depend on Ca 2+ transients in the ASH nociceptor neuron. Averaged Ca 2+ transients and a summary showing the respective Ca 2+ metric together with behavioral index for each mutant can be viewed in Figs 3 and 4 , and Supplementary Figs 3–5 . OSM-9 pore aromaticity is critical for ASH activation We sought to determine whether aromaticity is critical for Ca 2+ entry at positions Y 604 , Y 606 and F 609 . We did not observe a Ca 2+ response for any of the Y604F animals tested ( Fig. 3f ). A lack of Ca 2+ transients in Y604F animals, combined with rescue of the behavioral phenotype, suggests that Ca 2+ influx into ASH is dispensable for nocifensive behaviour, that another ion is contributing to OSM-9 function in activation of ASH ( Fig. 4b ), and that activation encompasses depolarization of the cell. Complimentary findings were recorded for Y606A, where we observed minimal Ca 2+ transients in 5/12 trials ( Fig. 3g and Supplementary Fig. 6I ) and complete absence thereof in 7/12. These transients were very shallow in comparison with the osm-9::gfp WT rescue and could only be visualized on a × 10 enlarged ordinate. Also, the transients displayed increased noise in comparison with a typical WT ASH transient, yet they did show proper ON/OFF peaks. For F609A, we did not observe any Ca 2+ transients, indicating that F 609 is a critical residue in ion permeation and selectivity ( Fig. 4b and Supplementary Figs 4F and 6L ). Divergence of Ca 2+ dynamics and rescue of osmotic avoidance Our combined results with Y604F and Y606A reiterate that in the absence of Ca 2+ influx or its strong reduction, appreciable osmotic avoidance behaviour can be elicited. In other words, in the absence of detectable Ca 2+ influx, ASH can be partially activated. When aromaticity is maintained, as in Y604F,differing by one –OH group, Ca 2+ influx changes from WT to non-detectable. At the same time, channel function ofY604F is sufficient to activate ASH and initiate the avoidance response, likely mediated by influx of an alternate cation, presumably sodium, resulting in ASH depolarization. We also tested mutants with partially defective behaviour. We observed no WT Ca 2+ transients in any of the trials for M601G, G602K and G603K ( Supplementary Fig. 5 ). Notably, G602K transients were the most variable ( Supplementary Figs 4D and 6D ). Ca 2+ transients were only observed in 7/14 trials, but none of those exhibited the typical ON/OFF peaks of normal Ca 2+ transients in ASH or were consistent in their defects. Many of the transients were delayed or failed to terminate after stimulus removal. These findings indicate that residues M 601 -G 602 -G 603 are critical for Ca 2+ influx into ASH, although they are not critical for activation of ASH. Determined efforts to obtain e-phys from the OSM-9 pore were unsuccessful ( Supplementary Note 2 ). ASH Ca 2+ dynamics drives behavioral plasticity In order to begin to understand the role of Ca 2+ that enters ASH upon OSM-9 activation in response to noxious osmotic cues, we conducted experiments that interrogate behavioral adaptation of the nocifensive response to repeated stimulation and to starvation. For both paradigms, we compared Y604F with WT rescue worms. We examined the adaptive response to repeat osmotic stimulation after extended exposure to hypertonicity ( Fig. 5a ). We found compelling evidence of lack of behavioral adaptation in Y604F worms. After exposure to hypertonic stimulus for 1 min, Y604F mutant worms avoided on average in at least 3/5 consecutive trials. In striking contrast, WT rescue worms avoided on average 1/5 trials, in keeping with the established desensitization after extended stimulation. In detail, there was no avoidance in any of the tested animals in trials 1/5 and 2/5. Y604F did not desensitize and showed avoidance with similar frequency throughout all five trials. Thus, worms lacking a detectable transient in ASH in response to noxious osmotic cues caused by the Y604F mutation do not desensitize as do OSM-9 WT rescue worms. Bespeaking of the specificity of this desensitization of osmotic avoidance, overexposure to octanol did not alter subsequent osmotic avoidance behaviour ( Fig. 5b ). OSM-9 WT rescue worms showed WT level osmotic avoidance, whereas Y604F animals displayed partial rescue. The altered sensory response to biogenic amines after starvation in Y604F mutant worms is shown in Fig. 5c and described in more detail in Supplementary Results . 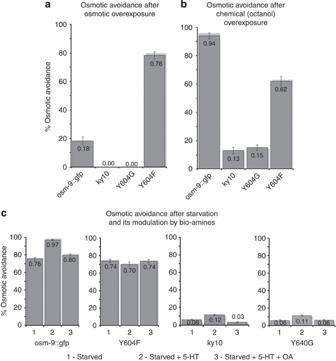Figure 5: Behavioral plasticity is diminished in Y604F mutant worms (a) Osmotic stimulus overexposure diminishes osmotic avoidance ofosm-9::gfpWT rescue worms, but not of Y604F mutants. Bars represent osmotic avoidance behaviour of the four tested worm strains represented on thexaxis. (b) Volatile chemical overexposure evokes no significant change in osmotic avoidance. Bars represent avoidance behaviour to octanol. (c) Response of starved worms to biogenic amines is altered in Y604F mutant worms. Bars in all panels represent osmotic avoidance behaviour. Note the expected increase of starved worms’ osmotic avoidance in response to serotonin (5-HT) exposure, reduction of this increase by addition of octopamine (OA) and lack of these responses in Y604F mutants. Bars represent mean, error bars s.e.m. ≥10 individual animals per line were tested, three lines for each strain. Figure 5: Behavioral plasticity is diminished in Y604F mutant worms ( a ) Osmotic stimulus overexposure diminishes osmotic avoidance of osm-9::gfp WT rescue worms, but not of Y604F mutants. Bars represent osmotic avoidance behaviour of the four tested worm strains represented on the x axis. ( b ) Volatile chemical overexposure evokes no significant change in osmotic avoidance. Bars represent avoidance behaviour to octanol. ( c ) Response of starved worms to biogenic amines is altered in Y604F mutant worms. Bars in all panels represent osmotic avoidance behaviour. Note the expected increase of starved worms’ osmotic avoidance in response to serotonin (5-HT) exposure, reduction of this increase by addition of octopamine (OA) and lack of these responses in Y604F mutants. Bars represent mean, error bars s.e.m. ≥10 individual animals per line were tested, three lines for each strain. Full size image Homology modelling helps illustrate the OSM-9 pore structure In order to generate a contemporary three-dimensional model of the OSM-9 pore that can function to illustrate the in vivo results presented here, we computationally modelled the closed conformation of the OSM-9 pore against templates of structurally resolved K + channels (crystallography) and TRPV1 (cryo-electron microscopy (EM); Supplementary Notes 3 and 4.1–4.8 ). Overall, our computational modelling data are in agreement with our in vivo results. In similar manner, several groups have generated homology models for the pore-forming region of TRPV1, TRPV3, TRPV6, TRPC3, TRPA1, TRPM4, Drosophila TRP and yeast TRPY1 (refs 1 , 43 , 53 , 54 , 55 ). These structural models have served as illustrations of the respective channels’ biophysics. We relied on structurally resolved potassium channels Kv1.2-2.1 Paddle Chimera Channel (PDB ID: 2R9R), the chicken inward-rectifier K + channel Kir2.2 (PDB ID: 3JYC) and TRPV1 cryo-EM structures (PDB ID: 3J5P) as templates [56] , [57] , [58] , [59] . Results are shown in Fig. 6 . More extensive descriptions and comments can be found in the Supplementary Information ( Supplementary Figs 8–15 , Supplementary Movie and Supplementary Data for pdb coordinates of the refined models). 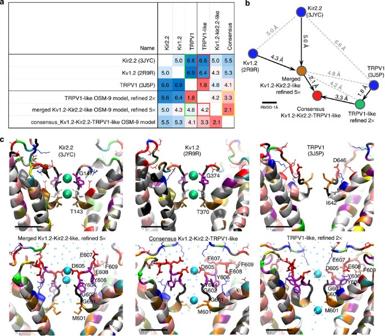Figure 6: Homology modelling, computational refining of the OSM-9 pore (a) Structural comparison of the starting crystallographic templates56,57,58,59and three refined homology models of OSM-9. Root mean square deviation (r.m.s.d. in Å) was calculated for the homologous regions covering TM helices S5 and S6, the pore helix and the selectivity filter (seeSupplementary Informationfor the details of the refinement process and more detailed r.m.s.d. table that includes the intermediate refinement stages). Refinement of Kir2.2-Kv1.2-based model makes it more similar to TRPV1 cryo-EM structure, comparing with the starting templates (green frames in the table). Refinement of the TRPV1-based model drives structure towards the Kv templates to certain extent and makes it more similar to the refined Kir2.2-Kv1.2-based model (red frames). Slow convergence of the refined Kir2.2-Kv1.2- and TRPV1-based models to a continuously updated average have produced a consensus model that is somewhat more similar to Kv- rather than TRPV1-based model (yellow frame). (b) A two-dimensional ‘map’ of the refinement process reflects pairwise structure similarity from r.m.s.d. table (a) as spatial proximity. (c) Snapshots of the selectivity filter in the starting template structures (top row) and the refined models (bottom row). Independent refinement of the Kv- (lower left) and TRPV1-based (lower right) models shows spontaneous coordination of the calcium ions by the acidic side chains rather than backbone that used to coordinate potassium ions in the crystallographic structures. Converging the refined models to a consensus structure leads to lengthening of the filter and formation of a stable ion-conducting water (cyan dots) pathway, similar to refined Kir2.2-Kv1.2-based model. Protein backbone is coloured by the residue name (Ala grey; Arg, Lys blue; Asn green; Asp, Glu red; Cys yellow; Gly black; Gln lime; His mauve; Ile, Leu white; Met orange; Phe pink; Pro cyan; Ser tan; Thr ochre; Trp, Tyr purple; and Val silver). Figure 6: Homology modelling, computational refining of the OSM-9 pore ( a ) Structural comparison of the starting crystallographic templates [56] , [57] , [58] , [59] and three refined homology models of OSM-9. Root mean square deviation (r.m.s.d. in Å) was calculated for the homologous regions covering TM helices S5 and S6, the pore helix and the selectivity filter (see Supplementary Information for the details of the refinement process and more detailed r.m.s.d. table that includes the intermediate refinement stages). Refinement of Kir2.2-Kv1.2-based model makes it more similar to TRPV1 cryo-EM structure, comparing with the starting templates (green frames in the table). Refinement of the TRPV1-based model drives structure towards the Kv templates to certain extent and makes it more similar to the refined Kir2.2-Kv1.2-based model (red frames). Slow convergence of the refined Kir2.2-Kv1.2- and TRPV1-based models to a continuously updated average have produced a consensus model that is somewhat more similar to Kv- rather than TRPV1-based model (yellow frame). ( b ) A two-dimensional ‘map’ of the refinement process reflects pairwise structure similarity from r.m.s.d. table ( a ) as spatial proximity. ( c ) Snapshots of the selectivity filter in the starting template structures (top row) and the refined models (bottom row). Independent refinement of the Kv- (lower left) and TRPV1-based (lower right) models shows spontaneous coordination of the calcium ions by the acidic side chains rather than backbone that used to coordinate potassium ions in the crystallographic structures. Converging the refined models to a consensus structure leads to lengthening of the filter and formation of a stable ion-conducting water (cyan dots) pathway, similar to refined Kir2.2-Kv1.2-based model. Protein backbone is coloured by the residue name (Ala grey; Arg, Lys blue; Asn green; Asp, Glu red; Cys yellow; Gly black; Gln lime; His mauve; Ile, Leu white; Met orange; Phe pink; Pro cyan; Ser tan; Thr ochre; Trp, Tyr purple; and Val silver). Full size image As qualifiers to this approach, we want to point out the relatively low homology of our templates (for S5 and S6 helices, 13.1% (Kir2.2), 12.3% (Kv1.2) and 26% (TRPV1)), which one has to bear in mind when appreciating results generated. It is important to acknowledge that for models that share <25% identity with their template structure, the analysis should be done extra carefully and the conclusions should be interpreted with caution. However, we also wish to point out that our models were refined via iterative cycles of a recently developed symmetry-restrained annealing protocol, which has been successfully tested in the molecular dynamic refinement of homology models of K+ channels [60] . Our homology models show a spontaneous convergence of the TRPV1-based and the K-channel based models ( Supplementary Fig. 14 and Supplementary Movie ). We have therefore generated a consensus model to reveal the most stable structural features [60] and also for illustrative purposes ( Fig. 6 and Supplementary Figs 10–15 ) Our modelling results indicate that the position of the filter relative to the pore stays stable even in simulations without cations in the vicinity of the selectivity filter. This increases confidence in our modelling. In addition, our approach suggests that the filter is compatible with both Ca 2+ and Na + ( Supplementary Fig. 12 and Supplementary Movie ), and that Y 604 could have a structurally stabilizing role ( Supplementary Note 5 ). The proposed higher position of D 605 in the selectivity filter of OSM-9 is in agreement with channel physiology experiments in TRPV4 (ref. 28 ). Results from this study suggested that TRPV4 D 682 , which aligns with OSM-9 D 605 , is likely to be in the outer region of the pore. Conservation of the selectivity filter in the TRPV family The OSM-9 sequence (SMGGYDYEEF) is more divergent from the mammalian TRPV1-4 sequence of TIG(M/L)G(D/E)LX(F/I/M) and TRPV5-6 sequence FLT(V/I)ID(A/G)PA, but negatively charged residues are found in both sequences, as are aromatic residues ( Fig. 7 ) [16] . The functional homologue of OSM-9, TRPV4, has a sequence of TIGMGDLEM in the mouse. Based on sequence analysis with additional invertebrate taxa, we found that the selectivity filter of a functionally related C. elegans TRPV channel, OCR-2, is TIGE F TVL Y RNL with F 721 and Y 725 aligning with OSM-9 Y 604 and Y 606 , respectively, over an insertion in the OCR-2 sequence. Notably, aromatics in the selectivity filter of OSM-9 resemble TRPV inactive (sequence in aphid TMGD Y N Y ADL) while OCR-2 resembles TRPV nanchung (sea squirt TLGE F QDL Y LDF). Intriguingly inactive and nanchung are functional partner ion channels, functional in insect hearing, similar to how OSM-9 and OCR-2 require each other [61] . 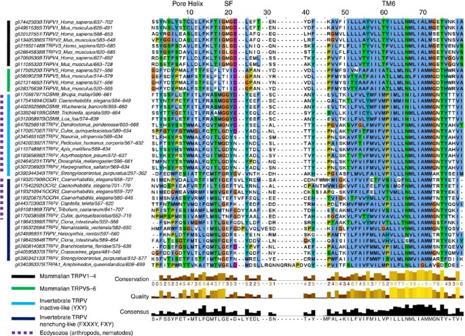Figure 7: Multiple sequence alignment elucidates evolutionary roots A multiple sequence alignment of 40 TRPV sequences from various mammalian and invertebrate taxa, plus 1 TRPA1 sequence from a marine sponge, used as an outgroup, was constructed for the pore helix to the end of TM6. The range of amino acids used for the alignment is denoted after the forward slash in the sequence name. Note that filters are variable in length, furthermore, both negatively charged and aromatic amino acid residues appear positioned for a critical role in the selectivity filter. Figure 7: Multiple sequence alignment elucidates evolutionary roots A multiple sequence alignment of 40 TRPV sequences from various mammalian and invertebrate taxa, plus 1 TRPA1 sequence from a marine sponge, used as an outgroup, was constructed for the pore helix to the end of TM6. The range of amino acids used for the alignment is denoted after the forward slash in the sequence name. Note that filters are variable in length, furthermore, both negatively charged and aromatic amino acid residues appear positioned for a critical role in the selectivity filter. Full size image Few studies have addressed the function of the selectivity filter of a TRPC in the context of a live organism. Here we present in vivo data on the selectivity filter of the C. elegans TRPV channel, OSM-9, showing that Ca 2+ is largely dispensable for nociceptor neuron activation that elicits nocifensive behaviour. Our data also support a concept that Ca 2+ is not dispensable for behavioral plasticity evoked by noxious stimulation. Furthermore, we demonstrate that aromatic and negatively charged residues are critical for selectivity filter function. Our computational modelling data provide possible structural interpretation with our in vivo results. Our in vivo mutational analysis, with additional guidance by computational assessments including structural modelling demonstrates that the invertebrate TRPV channel, OSM-9, contains a predicted ion selectivity filter directly C-terminal to the pore helix, and that its boundaries extend from M 601 -F 609 . We found that mutation of these residues disrupts channel function in the live organism. This conclusion is based on assessment of avoidance behaviour, Ca 2+ imaging and subcellular expression studies of the transgenic channels in the primary sensory neuron, ASH, a nociceptor neuron in which OSM-9 is expressed. Specifically, we found that residues Y 604 , D 605 and F 609 are critical for activation of and Ca 2+ entry into ASH. Negatively charged residues are found in selectivity filters of ion channels that conduct cations, and have been determined to be critical for ion selectivity and permeation in TRPCs [16] , [62] . A study focusing on D 621 of the Drosophila TRPC selectivity filter showed that this residue is critical for Ca 2+ permeability in fly photoreceptors and is a pore-lining residue [38] . Ca 2+ influx through dTRP was found to be significant for phototransduction and photoreceptor survival. Thus, when comparing fly phototransduction and worm osmotic avoidance behaviour, the roles of TRPC-mediated Ca 2+ influx are not identical, in that Ca 2+ is essential for phototransduction, but dispensable for nocifensive behaviour. The only other study to characterize a TRPC selectivity filter in vivo focused on the C. elegans TRPN mechanotransduction channel, trp-4 (ref. 39 ). Again, the authors evaluated negatively charged residues and found that two residues C-terminal to the pore helix, E 1739 and D 1741 , are critical for activation of the CEP sensory neuron in response to changes of external viscosity. Thus, our finding that D 605 and E 607 are critical for behaviour is in keeping with this study. Notably, both TRP-4 and OSM-9 have important negatively charged residues separated by one amino acid in the heart of the selectivity filter. The CEP neuron was assessed by patch-clamp recordings but Ca 2+ signalling was not analysed in this study [39] . Both of these elegant in vivo studies have focused on negatively charged residues and identified the ones critical for selectivity. Our systematic deconstruction of the OSM-9 selectivity filter using behavioral analysis of nocifensive behaviour, in vivo Ca 2+ imaging, expression studies in ASH and molecular dynamic simulations of channel structure mirrors previous findings and provides additional new mechanistic insight. Our findings suggest that depolarization of the primary nociceptor neuron via influx of Na + can be sufficient as a critical driving force to elicit nocifensive behaviour. In addition, our experiments to elucidate behavioral plasticity drive home the point that Ca 2+ influx via TRPV channels is a critical component of neurosensory transduction that leads to an adaptive behavioral response to subsequent stimuli or in situations of altered environmental stress such as starvation. This insight, now rooted in experimental data, has relevance for evolution of pain signalling, discussed more below. But it also might serve as an incentive to isolate novel TRP channel-specific antagonist compounds, for treatment of pain and also other medically relevant conditions, that are Ca 2+ selective and rather leave Na + unaffected. Finally, we examine our findings in the context of nociceptor evolution. Previous studies have shown that TRPV4 can rescue the defects of osm-9 null mutants in sensing of noxious osmotic and mechanical cues [29] . The role of TRPV4 in nociception is well established in response to noxious mechanical stimuli (without sensitization) in inflammation, and nerve-and tissue damage [5] , [7] , [15] . The evolution of mammalian pain sensing can also be traced ancestrally to the TRPCs of Drosophila [63] . Since we have investigated the function of the selectivity filter of OSM-9 in the context of avoidance behaviour in response to noxious cues, our present results can therefore be viewed as informative for the evolution of pain signalling. Specifically, the finding that Ca 2+ is dispensable for activation of the nociceptor neuron, ASH, adds a new dimension to our understanding of this critical process in pain signalling. We find it exciting to speculate that cationic selectivity of TRP(V) channels in nociceptors has been shaped by evolution so that these channels conduct Ca 2+ preferentially over Na + in order to regulate the neurosensory cell’s plasticity in response to subsequent stimulation. This attractive concept is supported by our data set on behavioral plasticity. This in turn could possibly indicate that transduction of noxious cues by TRP ion channels has an inbuilt mechanism to adapt the organism to future challenges. This is an advantageous mechanism in terms of organismal and species survival when compared with simple nociceptor activation by Na + or indiscriminate cationic influx. However, we did not study how the Ca 2+ -mediated adaptive response affects nociceptor gene regulation, a longer-term and more permanent regulatory mechanism. This will be a worthy subject for future studies. Strains and genetics The N2 (Bristol) isolate of C. elegans was used for all experiments. Strains were maintained and manipulated under standard conditions as described [64] . Analyses were performed at 25 °C unless otherwise noted [64] . Strains and transgenes used in this work were. LGIV osm-9(ky10); transgenes: aslEx001[sra-6::gfp]; aslEx003[psra-6::osm-9::gfp]; aslEx016[psra-6::Δ601-619::gfp]; aslEx025[psra-6::Δ601-606::gfp]; aslEx026[psra-6::Δ604-609::gfp]; aslEx027[psra-6::Δ607-612::gfp]; aslEx028[psra-6::Δ610-615::gfp]; aslEx029[psra-6::Δ613-619::gfp]; aslEx042[psra-6::M601G::gfp]; aslEx063[psra-6::G602K::gfp]; aslEx064[psra-6::G603K::gfp]; aslEx041[psra-6::Y604G::gfp]; aslEx051[psra-6::Y604E::gfp]; aslEx052[psra-6::Y604F::gfp]; aslEx065[psra-6::D605K::gfp]; aslEx010[psra-6::Y606A::gfp]; aslEx077[psra-6::E607A::gfp]; aslEx078[psra-6::E608A::gfp]; aslEx079[psra-6::F609A::gfp]; aslEx040[psra-6::Y614A::gfp];aslEx042[psra-6::M601G::gfp)/kyEx2865[psra-6::G-CaMP3], aslEx063[psra-6::G602K::gfp)/kyEx2865[psra-6::G-CaMP3], aslEx064[psra-6::G603K::gfp]/ kyEx2865[psra-6::G-CaMP3], aslEx041[psra-6::Y604G::gfp]/ kyEx2865[psra-6::G-CaMP3], aslEx052[psra-6::Y604F::gfp]/kyEx2865[psra-6::G-CaMP3], aslEx065[psra-6::D605K::gfp]/kyEx2865[psra-6::G-CaMP3], aslEx010[psra-6::Y606A::gfp]/kyEx2865[psra-6::G-CaMP3]; aslEx077[psra-6::E607A::gfp]/kyEx2865[psra-6::G-CaMP3]; aslEx078[psra-6::E608A::gfp]/kyEx2865[psra-6::G-CaMP3]; aslEx079[psra-6::F609A::gfp]/kyEx2865[psra-6::G-CaMP3]; aslEx040[psra-6::Y614A::gfp]/kyEx2865[psra-6::G-CaMP3]; aslEx081 [ocr-2::tdT/egl-15::gfp]; aslEx082 [ocr-2::tdT/rol-6]; aslEx041 [psra-6::Y604G::gfp]/aslEx081 [ocr-2::tdT/egl-15::gfp]; aslEx041 [psra-6::Y604G::gfp]/aslEx082 [ocr-2::tdT/rol-6]; aslEx052[psra-6::Y604F::gf]/aslEx081 [ocr-2::tdT/egl-15::gfp]; aslEx052[psra-6::Y604F::gfp]/aslEx082 [ocr-2::tdT/rol-6]; aslEx065 [psra-6::D605K::gfp]/aslEx081 [ocr-2::tdT/egl-15::gfp]; aslEx065 [psra-6::D605K::gfp]/aslEx082 [ocr-2::tdT/rol-6]; aslEx010 [psra-6::Y606A::gfp]/aslEx081 [ocr-2::tdT/egl-15::gfp]; aslEx010 [psra-6::Y606A::gfp]/aslEx082 [ocr-2::tdT/rol-6]; aslEx040 [psra-6::Y614A::gfp]/aslEx081 [ocr-2::tdT/egl-15::gfp]; aslEx040 [psra-6::Y614A::gfp]/aslEx082 [ocr-2::tdT/rol-6]. Generation of transgenic animals Adult animals were injected with 50–150 ng μl −1 of construct DNA and vha-6 ::red fluorescent protein (RFP) intestinal marker at 70 ng μl −1 . Transgenic animals were selected and maintained as stable lines [65] . All transgenic animals were characterized for five generations to establish the stability of the line before behavioral assays were conducted. Individual behavioral assays Tests were performed with investigators blinded to genotype [40] . In brief, 1–2 μl of 1 M fructose were dropped from a drawn capillary tube into the path of a forward-moving worm. After coming into contact with the drop, WT worms reverse the direction of movement and withdraw from the drop within 2 s. Avoidance defective worms do not reverse the direction, but continue to move through the drop. Animals are videotaped and the video is analysed for percent of response. Behavioral avoidance is assessed by testing three lines for each strain, 10 animals each, on 2 different days, to give six sample sets of population data. Results are averaged and presented as Avoidance Index. Avoidance Index is defined by normalization to osm-9::gfp WT rescue and then osm-9( ky10) results for the day of testing. For examination of behavioral plasticity, worms were exposed for 1 min to 1 M fructose or volatile exposure to 30% octanol, and subsequently stimulated 5 × by osmotic drop test, as described above. The interstimulus interval was 10 s. Starvation, 5-HT and octopamine exposure were conducted by starving the worms for 24 h on bacteria-free plates, and using 5-HT and octopamine at 4 mM (refs 66 , 67 , 68 ). Mechanical avoidance assays Nose touch was analysed as described previously [69] . In brief, six animals from each of three lines were scored 10 times, at two different time points, and the results were averaged to obtain percent avoidance for each strain. Volatile chemical avoidance assays Aversive odorant sensing was analysed as described previously using 10% octanol [29] . In brief, six animals from each of three lines were scored five times, at two different time points, and the results were averaged to obtain percent avoidance for each strain. Molecular biology The StratageneQuikChange XL Site-Directed Mutagenesis Kit was used to generate amino acid deletions and exchanges to produce separate, C-terminally GFP-tagged osm-9 cDNA constructs. Details of plasmid construction are available upon request. Confocal microscopy Worms were mounted on 2% agar pads and paralysed with 150 mM levamisole-HCl. Confocal images with bright field were obtained using a Zeiss LSM510 microscope using a × 40/1.3 numerical aperture oil immersion objective. Z-stacks and projections were generated using the Zeiss 5Live Imaging software. Delta imaging system Worms were mounted on 2% agar pads and paralysed with 150 mM levamisole-HCl. Worms were examined using an Olympus IX-71 microscope using a × 60/1.42 numerical aperture oil immersion objective. Images were collected using 488 nm laser lines for excitation and GFP 525/50 and mCherry 632/60 emission filters. An Evolve back-thinned EM-CCD camera (512 × 512) was used to capture images, and Z-stacks were acquired with an interval of 0.25–0.4 μm, and the gain and offset were optimized for the brightest central planes of the stack. SoftWoRx 5.0, with system-level queuing, was used to process images Ca 2+ imaging in live worms Imaging was performed as previously described [43] . In brief, worms for each genotype were studied in a multi-chambered microfluidics device that restrains individual animals while exposing the worm nose to a soluble stimulus. Worms were generated by mating a characterized line of sra-6::G-CaMP3 to the osm-9 mutant transgenic line most representative of the average behavioral response for that mutation. Fluorescence levels from the Ca 2+ indicator protein G-CaMP3 were measured for each worm and were averaged. Worms were first loaded into the chip and then were bleached for 70 s to remove the ASH-induced ultraviolet light response. A quantity of 1 M fructose was then presented at t =10 s and removed at t =40 s, the total recording time was 70 s. Animals (12–16) were each tested once for individual mutant strains, and the resulting Ca 2+ transients were averaged to determine the Ca 2+ activity in ASH for that mutation. Non-normal data sets were not averaged and are displayed as raw data. Computational modelling of OSM-9 Methods for homology modelling and molecular dynamic refinement of the closed conformation of OSM-9 are described in Supplementary Information . How to cite this article: Lindy, A. S. et al. TRPV channel-mediated calcium transients in nociceptor neurons are dispensable for avoidance behaviour. Nat. Commun. 5:4734 doi: 10.1038/ncomms5734 (2014).